The deubiquitinating enzyme USP17 is essential for GTPase subcellular localization and cell motility Deubiquitinating enzymes are now emerging as potential therapeutic targets that control many cellular processes, but few have been demonstrated to control cell motility. Here, we show that ubiquitin-specific protease 17 (USP17) is rapidly and transiently induced in response to chemokines SDF-1/CXCL12 and IL-8/CXCL8 in both primary cells and cell lines, and that its depletion completely blocks chemokine-induced cell migration and cytoskeletal rearrangements. Using live cell imaging, we demonstrate that USP17 is required for both elongated and amoeboid motility, in addition to chemotaxis. USP17 has previously been reported to disrupt Ras localization and we now find that USP17 depletion blocks chemokine-induced subcellular relocalization of GTPases Cdc42, Rac and RhoA, which are GTPases essential for cell motility. Collectively, these results demonstrate that USP17 has a critical role in cell migration and may be a useful drug target for both inflammatory and metastatic disease. The post-translational modification of proteins through ubiquitination is critical for proper regulation of numerous intracellular processes. Consequently, removal of ubiquitin from these modified proteins by deubiquitinating enzymes (DUBs) is also vital, and a growing body of evidence shows that these enzymes are essential for regulation of many cellular functions including transcription, DNA repair, cell-cycle progression and apoptosis [1] , [2] , [3] . The ubiquitin-specific protease 17 (USP17) is an immediate early gene that belongs to a subfamily of cytokine-inducible DUBs. The murine members of this family were initially identified as cytokine-inducible genes [4] , [5] , [6] , [7] , as is the human orthologue USP17 (ref. 8 ). Specifically, USP17 is induced by IL-4 and IL-6, which regulate the growth and differentiation of leukocytes [8] . More recently, we have demonstrated that USP17 controls the function of the small GTPase Ras through abrogation of its post-translational processing and membrane localization [9] , [10] . We, along with others, have also postulated that USP17 regulates the cell cycle at G1/S phase, thus regulating cell proliferation [11] , [12] . Chemotaxis, or cell migration, is an important cellular function in multicellular organisms for normal homeostasis and development, but it is frequently deregulated in disease states such as inflammation and metastatic cancer progression [13] , [14] . Two types of cell migration have been identified: mesenchymal (wherein cells are elongated and form focal adhesions) [15] , [16] and amoeboid (wherein cells have a blebbing/rounded morphology, transient adhesions and increased velocity) [17] , [18] . The Rho family of GTPases, through cycling between the inactive GDP and active GTP state, has a predominant role in regulating these processes [14] , [19] . Their activation at the plasma membrane initiates signalling cascades and the control of cytoskeletal dynamics. RhoA activity is elevated in blebbing cells and indeed localizes to the bleb-like protrusions [20] , whereas mesenchymal migration is characterized by Rac1 activation and decreased downstream activation of LIM kinase [21] , [22] . In addition, Cdc42 can induce both modes of migration [23] , [24] . As cells are able to alter their morphology and mode of migration depending on their environment, regulation of these processes is critical. Therefore, by inhibiting both mesenchymal and amoeboid migration, this may be a point of putative therapeutic intervention for diseases such as metastatic cancer and inflammation. As the Rho family of GTPases is known to be involved in migration, and USP17 was shown to control Ras plasma membrane localization [10] , we postulated that USP17 would similarly affect Rho GTPase localization and cell motility. Here, we show chemokine regulation of this DUB in both elongated and amoeboid motility. Moreover, we demonstrate that USP17 depletion blocks normal cytoskeletal rearrangements and chemokine-induced membrane localization of Rho GTPases. Therefore, USP17 is essential for the relocalization of Rho GTPases during normal cell motility. USP17 is a chemokine-inducible gene essential for chemotaxis As USP17 has previously been shown to be inducible upon cytokine stimulation, we first examined whether USP17 was induced in response to chemokines ( Fig. 1 ). We found that USP17 expression was rapidly and transiently induced in human peripheral blood mononuclear cells (PBMCs) following stimulation with CXCL12 ( Fig. 1a,b ). At 30 min after stimulation, mRNA levels increased dramatically, returning to baseline at 90 min ( Fig. 1a ), when the most prominent increase in protein levels was detected ( Fig. 1b ). Similar USP17 upregulation was observed in HeLa ( Fig. 1c,d ) and Jurkat T cells ( Fig. 1e ). However, USP17 upregulation was more rapid in both HeLa and Jurkat cells than in PBMCs, perhaps because PBMCs are a mixture of cell types of which only some respond to CXCL12. In addition, USP17 expression was also increased in neutrophils ( Fig. 1f ) and the human monocytic cell line U937 ( Fig. 1g ) when stimulated with CXCL8/IL-8. These results implied that USP17 may have an important role in inducing the chemotactic response in primary cells and in cell lines. 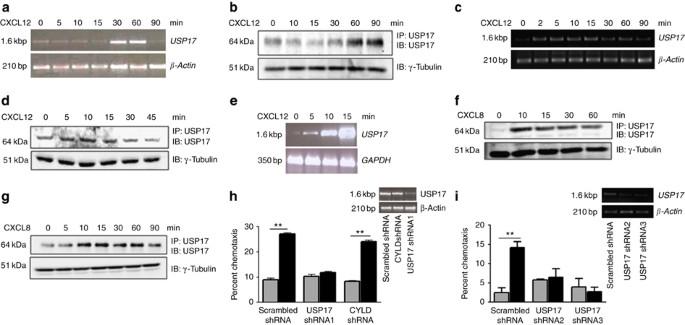Figure 1: USP17 expression is required for chemotaxis. Human PBMCs (a,b) or HeLa cells (c,d) were stimulated with CXCL12 (100 ng ml−1) for the indicated times.USP17mRNA expression was assessed by RT–PCR (a,c) and USP17 protein was determined by immunoprecipitation (IP), followed by immunoblotting (IB) (b,d). In mRNA images,β-actinwas used as a loading control, whereas γ-tubulin was the control for western blotting. (e) Jurkat T cells were serum starved and then stimulated with CXCL12 (100 ng ml−1) for 0, 5, 10 and 15 min. USP17 mRNA was analysed by RT–PCR. glyceraldehyde 3-phosphate dehydrogenase (GAPDH) mRNA was also analysed as a loading control. Human neutrophils extracted from blood (f) or the monocytic cell line U937 (g) were stimulated with CXCL8 (100 ng ml−1) for the indicated times. USP17 protein was immunoprecipitated then blotted for USP17. Whole-cell lysates were analysed for γ-tubulin as a loading control. (h,i) HeLa cells were transfected with either scrambled shRNA, USP17 shRNA1 or CYLD shRNA (h) or scrambled and two additional shRNAs targeting USP17 (shRNA2 and shRNA3) (i). Cells were left unstimulated (grey bars) or stimulated with CXCL12 (20 ng ml−1) (black bars) and chemotaxis was measured in modified Boyden chambers. RT–PCR was used to determineUSP17mRNA expression andβ-actinwas used as a loading control. Experiments were conducted in triplicate; values are mean±s.e.m.; and statistical analyses are relative to untreated control by one-way analysis of variance. **P>0.05. Figure 1: USP17 expression is required for chemotaxis. Human PBMCs ( a , b ) or HeLa cells ( c , d ) were stimulated with CXCL12 (100 ng ml −1 ) for the indicated times. USP17 mRNA expression was assessed by RT–PCR ( a , c ) and USP17 protein was determined by immunoprecipitation (IP), followed by immunoblotting (IB) ( b , d ). In mRNA images, β-actin was used as a loading control, whereas γ-tubulin was the control for western blotting. ( e ) Jurkat T cells were serum starved and then stimulated with CXCL12 (100 ng ml −1 ) for 0, 5, 10 and 15 min. USP17 mRNA was analysed by RT–PCR. glyceraldehyde 3-phosphate dehydrogenase ( GAPDH ) mRNA was also analysed as a loading control. Human neutrophils extracted from blood ( f ) or the monocytic cell line U937 ( g ) were stimulated with CXCL8 (100 ng ml −1 ) for the indicated times. USP17 protein was immunoprecipitated then blotted for USP17. Whole-cell lysates were analysed for γ-tubulin as a loading control. ( h , i ) HeLa cells were transfected with either scrambled shRNA, USP17 shRNA1 or CYLD shRNA ( h ) or scrambled and two additional shRNAs targeting USP17 (shRNA2 and shRNA3) ( i ). Cells were left unstimulated (grey bars) or stimulated with CXCL12 (20 ng ml −1 ) (black bars) and chemotaxis was measured in modified Boyden chambers. RT–PCR was used to determine USP17 mRNA expression and β-actin was used as a loading control. Experiments were conducted in triplicate; values are mean±s.e.m. ; and statistical analyses are relative to untreated control by one-way analysis of variance. ** P >0.05. Full size image Therefore, to explore the importance of this DUB in chemokine-induced cell migration, scrambled small hairpin RNA (shRNA) or USP17 shRNA1-transfected HeLa cells were stimulated with CXCL12, and migration was analysed using the modified Boyden chamber assay. USP17 depletion consistently ablated CXCL12-stimulated chemotaxis to levels equivalent to unstimulated cells, whereas an alternative shRNA targeting another DUB termed CYLD had no effect on chemotaxis ( Fig. 1h ), highlighting specificity for the role of USP17. Two additional USP17 shRNAs (USP17 shRNA2 and shRNA3) similarly reduced chemotaxis ( Fig. 1i ). Markedly reduced chemotaxis was also observed in MDA-MB-231 and U937 cells ( Supplementary Fig. S1a and b , respectively). USP17 depletion by reverse transcription PCR (RT–PCR) is also illustrated. Moreover, overexpression of USP17 further enhances chemotaxis in MDA-MB-231 cells ( Supplementary Fig. S1c ). Taken together, these data demonstrated that USP17 is required for directional migration. To exclude the possibility that USP17 affects chemokine receptor levels, we also examined the CXCL12 receptor, CXCR4, in HeLa cells and observed equivalent surface expression in the presence of USP17 shRNA1 or scrambled shRNA ( Supplementary Fig. S2a ). We further examined the external versus internal pools of CXCR4 and again observed no significant difference between scrambled and USP17 shRNA1-transfected cells ( Supplementary Fig. S2b ). Therefore, these finding clearly indicate that USP17 functions downstream of the receptor. USP17 expression is also required for chemokinesis In addition to chemotactic movement, cells can also migrate in a random undirectional manner, termed chemokinesis [25] . Therefore, to establish whether USP17 expression was also essential for chemokinesis, the migration of Hut78 T cells, either transfected with scrambled or USP17 shRNA1 bicistronic EGFP-expressing vectors, was examined. The cells were plated into wells coated with an antibody to the integrin leucocyte function associated-1 and images were captured over 90 min at 60 s intervals. USP17-depleted cells displayed a more rounded morphology and migration was decreased ( Fig. 2a , Supplementary Movies 1 and 2 ). In triplicate experiments, quantification of Hut78 T cells with depleted USP17 showed >50% reduced chemokinesis (as well as decreased cell velocity) when compared with scrambled control ( Fig. 2b,c ). Therefore, USP17 expression is not only required for chemokine-induced directional migration but also for random cell motility. 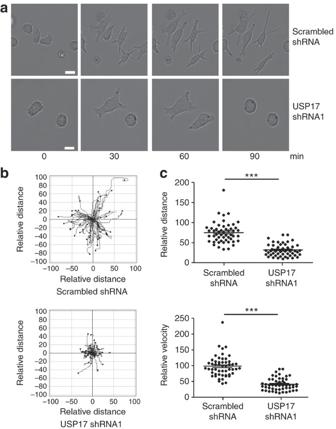Figure 2: USP17 depletion inhibits chemokinesis. Hut78 T cells were cotransfected with either scrambled shRNA or USP17 shRNA1 together with pMAX-GFP to determine transfected cells. Cells were allowed to adhere to culture plates coated with a CD11a/leucocyte function associated-1 antibody for 15 min before image acquisition using the IN Cell Imager. Brightfield images were captured every 60 s for 90 min; fluorescent images at 488 nM were captured at 0 and 90 min to confirm transfection. Scale bar, 20 μm. (a) Representative images of cells at 0, 30, 60 and 90 min (scale bar, 20 μm). (b) Cell trajectories where each line indicates an individual cell's migration. (c) A total of 60 cells were scored for distance and velocity and shown graphically. Each point represents one track, and the bar displays the median value. ***P>0.005 as determined by one-way analysis of variance. Figure 2: USP17 depletion inhibits chemokinesis. Hut78 T cells were cotransfected with either scrambled shRNA or USP17 shRNA1 together with pMAX-GFP to determine transfected cells. Cells were allowed to adhere to culture plates coated with a CD11a/leucocyte function associated-1 antibody for 15 min before image acquisition using the IN Cell Imager. Brightfield images were captured every 60 s for 90 min; fluorescent images at 488 nM were captured at 0 and 90 min to confirm transfection. Scale bar, 20 μm. ( a ) Representative images of cells at 0, 30, 60 and 90 min (scale bar, 20 μm). ( b ) Cell trajectories where each line indicates an individual cell's migration. ( c ) A total of 60 cells were scored for distance and velocity and shown graphically. Each point represents one track, and the bar displays the median value. *** P >0.005 as determined by one-way analysis of variance. Full size image USP17 is required for mesenchymal and amoeboid migration As previously outlined, cells can undergo either mesenchymal or amoeboid migration. As USP17 depletion resulted in decreased chemokinesis, we next examined whether both forms of migration were being inhibited. In scrambled shRNA-transfected cells, the majority of cells were elongated, displayed a leading edge and a tail and, following chemokine stimulation, were able to migrate ( Fig. 3a,b and Supplementary Movies 3 and 4 ). However, most USP17-depleted cells, did not form projections but instead produced blebs on the periphery of the cell ( Fig. 3c,d and Supplementary Movies 5 and 6 ). An additional shRNA against USP17 (USP17 shRNA2) induced the same changes in morphology, whereas CYLD shRNA cells appeared unaffected, similar to scrambled shRNA cells ( Supplementary Fig. S3 ). RT–PCR analysis on USP17 mRNA was performed to confirm USP17 depletion compared with β-actin control ( Fig. 3e and Supplementary Fig. S3e ). The apparent alteration in cell shape was not as obvious in fixed cells, as those cells with a rounded morphology would have decreased adhesions and would be washed off during preparation. Crucially, however, following chemokine stimulation, USP17-silenced cells have decreased migration ( Fig. 2 ). This suggests that depleting cells of USP17 blocks the cytoskeletal changes required for both elongated and amoeboid migration. 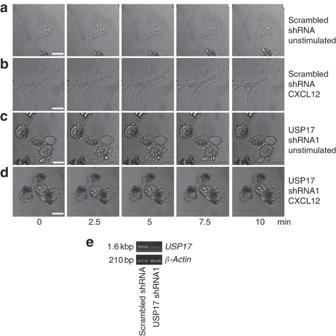Figure 3: USP17 shRNA alters cell morphology. HeLa cells transfected with scrambled shRNA were left unstimulated (a) or stimulated with CXCL12 (100 ng ml−1) (b). USP17 shRNA1 cells were unstimulated (c) or stimulated with CXCL12 (100 ng ml−1) (d). Brightfield images were captured every 15 s for 10 min by time-lapse microscopy using Leica SP5. Representative images from triplicate experiments are shown. Scale bar, 20 μm. (e) RT–PCR was used to confirm USP17 depletion using mRNA from HeLa cells by examiningUSP17andβ-actinmRNA expression. Figure 3: USP17 shRNA alters cell morphology. HeLa cells transfected with scrambled shRNA were left unstimulated ( a ) or stimulated with CXCL12 (100 ng ml −1 ) ( b ). USP17 shRNA1 cells were unstimulated ( c ) or stimulated with CXCL12 (100 ng ml −1 ) ( d ). Brightfield images were captured every 15 s for 10 min by time-lapse microscopy using Leica SP5. Representative images from triplicate experiments are shown. Scale bar, 20 μm. ( e ) RT–PCR was used to confirm USP17 depletion using mRNA from HeLa cells by examining USP17 and β-actin mRNA expression. Full size image USP17 depletion blocks cytoskeleton rearrangements As USP17 knockdown inhibited cell migration, and cytoskeletal reorganization is intricately involved in cell polarization and movement, we examined actin and tubulin polymerization as a potential mechanism. HeLa cells were transfected with scrambled shRNA or USP17 shRNA1, stimulated with CXCL12 and subsequently stained with α-tubulin (green) and phalloidin (red; detecting tubulin and actin polymerization, respectively) to visualize membrane ruffling and leading edge formation. Following stimulation, control cells displayed clear membrane ruffles (white arrow) indicative of lamellipodial or leading edge formation, whereas USP17-depleted cells showed decreased actin and tubulin polymerization and markedly reduced ruffling ( Fig. 4a ). Membrane ruffling was quantified 2 and 5 min after treatment in scrambled, USP17 and CYLD shRNA-transfected cells and shown graphically, confirming that USP17 was required ( Fig. 4b and Supplementary Fig. S4 ). USP17 shRNA2 also displayed similar results such that little actin polymerization was observed after chemokine stimulation ( Supplementary Fig. S4 ). Results from triplicate experiments clearly indicated that depletion of USP17 blocks chemokine-dependent cytoskeletal reorganization during lamellipodia formation, and that this effect was specific for USP17 and not for DUBs in general. 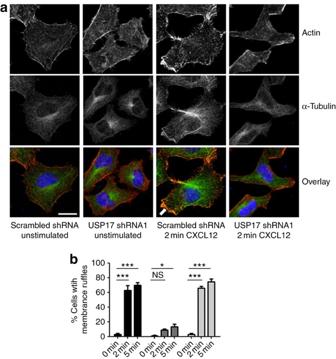Figure 4: USP17 depletion inhibits cytoskeleton rearrangements. HeLa cells were transfected with scrambled shRNA or USP17 shRNA1, and stimulated with CXCL12 (100 ng ml−1) for 0, 2 or 5 min. (a) Cells were costained for actin-phalloidin (red), α-tubulin (green) and 4,6-diamidino-2-phenylindole (blue) and representative images captured by the Leica SP5 microscope. Arrows depict membrane ruffles; scale bar, 20 μm. (b) Quantification of membrane ruffles of triplicate experiments is represented graphically. Black bars are scrambled shRNA-, dark grey bars are USP17 shRNA1- and light grey are CYLD shRNA-transfected cells. Values are mean±s.e.m. ***P>0.005, *P>0.01; NS, not significant as determined by analysis of variance. Figure 4: USP17 depletion inhibits cytoskeleton rearrangements. HeLa cells were transfected with scrambled shRNA or USP17 shRNA1, and stimulated with CXCL12 (100 ng ml −1 ) for 0, 2 or 5 min. ( a ) Cells were costained for actin-phalloidin (red), α-tubulin (green) and 4,6-diamidino-2-phenylindole (blue) and representative images captured by the Leica SP5 microscope. Arrows depict membrane ruffles; scale bar, 20 μm. ( b ) Quantification of membrane ruffles of triplicate experiments is represented graphically. Black bars are scrambled shRNA-, dark grey bars are USP17 shRNA1- and light grey are CYLD shRNA-transfected cells. Values are mean±s.e.m. *** P >0.005, * P >0.01; NS, not significant as determined by analysis of variance. Full size image USP17 is required for the membrane localization of GTPases To further study the mechanism by which USP17 regulates cell migration, the localization of the Rho family of small GTPases was examined. Rho GTPases have a central role in the regulation of cell migration through remodelling of the cytoskeleton. We have previously implicated USP17 as a key regulator of GTPases Ras and RhoA in cell proliferation [11] . In addition, mesenchymal and amoeboid migration are differentially regulated by the Rho family of GTPases; RhoA has been demonstrated to induce blebbing, whereas Rac1 regulates elongated movement, and Cdc42 can induce both morphologies [26] . Therefore, we assessed the effect of USP17 depletion on the intracellular localization and activation of Rac1, RhoA and Cdc42 in the context of cell migration. In unstimulated cells, these GTPases are localized primarily to the cytosolic regions of the cells. Following CXCL12 stimulation in control scrambled shRNA cells, the GTPases are transported to the plasma membrane ( Fig. 5a–c white arrows). However, in USP17-depleted cells (shRNA1), the plasma membrane localization of Cdc42, Rac1 and RhoA was markedly blunted ( Fig. 5a–c , respectively). In addition, USP17 shRNA2 also resulted in a mislocalization of RhoA, whereas CYLD shRNA had no effect on its transport ( Supplementary Fig. S5 ). The localization of endogenous RhoA, Cdc42 and Rac1 was also examined and a similar trend was observed such that USP17 was required for GTPase membrane localization following chemokine stimulation ( Supplementary Fig. S6 ). Fluorescent images were overlayed on brightfield images to confirm that the endogenous GTPases were indeed localized to the plasma membrane area, specifically in membrane ruffles (white arrows). 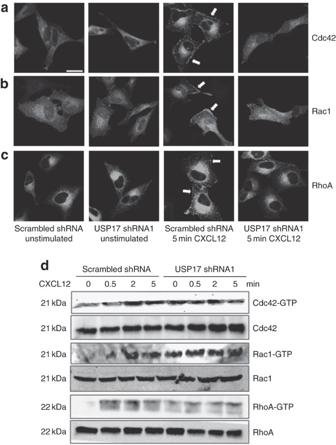Figure 5: Knockdown of USP17 inhibits GTPase localization and activation. HeLa cells were transfected with scrambled shRNA or USP17 shRNA1 along with GFP-tagged Cdc42 (a), Rac1 (b) and RhoA (c). Cells were either left unstimulated or stimulated with CXCL12 (100 ng ml−1) for 5 min and captured by confocal microscopy (Leica SP5). Arrows indicate sites of plasma membrane localization. Scale bar, 20 μm. (d) Cells were transfected as ina–c, stimulated with CXCL12 (100 ng ml−1) for 0, 0.5, 2 or 5 min and analysed for GTPase activation by performing pulldown assays for the indicated GTPase. Pulldowns and whole-cell lysates were immunoblotted with Cdc42, Rac1 or RhoA antibodies as indicated. Data shown are representative of three experiments. Figure 5: Knockdown of USP17 inhibits GTPase localization and activation. HeLa cells were transfected with scrambled shRNA or USP17 shRNA1 along with GFP-tagged Cdc42 ( a ), Rac1 ( b ) and RhoA ( c ). Cells were either left unstimulated or stimulated with CXCL12 (100 ng ml −1 ) for 5 min and captured by confocal microscopy (Leica SP5). Arrows indicate sites of plasma membrane localization. Scale bar, 20 μm. ( d ) Cells were transfected as in a – c , stimulated with CXCL12 (100 ng ml −1 ) for 0, 0.5, 2 or 5 min and analysed for GTPase activation by performing pulldown assays for the indicated GTPase. Pulldowns and whole-cell lysates were immunoblotted with Cdc42, Rac1 or RhoA antibodies as indicated. Data shown are representative of three experiments. Full size image Recruitment of Rho GTPases to the plasma membrane allows them to interact with their respective GEFs, resulting in their activation and downstream signalling. Therefore, GTPase activation was also examined by GST-Rhotekin and GST-PAK pulldown assays ( Fig. 5d ). In scrambled shRNA-transfected cells, we observed increased Cdc42, Rac1 and RhoA activation following CXCL12 stimulation ( Fig. 5d ). However, in USP17-depleted cells, basal constitutive GTPase activation was detected before stimulation and CXCL12 did not induce any detectable response ( Fig. 5d ). Again, USP17 shRNA2 yielded similar results to USP17 shRNA1, whereas CYLD shRNA did not alter RhoA activation ( Supplementary Fig. S7 ). It is well documented that these GTPases are localized to membrane ruffles of migrating cells [27] . Indeed, we observed Cdc42 and RhoA localization at these sites along with actin filaments following CXCL12 stimulation in control cells ( Fig. 6a,b ). Not surprisingly, in USP17-depleted cells, Cdc42 and RhoA were not localized to the edge of the cells, and no increase in short actin fibres, indicative of ruffling, was observed. Thus, USP17 is required for the proper localization of these GTPases to the leading edge and subsequent migration. We further confirmed that RhoA membrane localization was disrupted in USP17-depleted cells using total internal reflective fluorescence (TIRF), which allows selective detection of proteins specifically at the plasma membrane in living cells ( Fig. 6c ). Thus, these TIRF data add to the confocal data, demonstrating that USP17 is required for the localization of GTPases to the membrane. 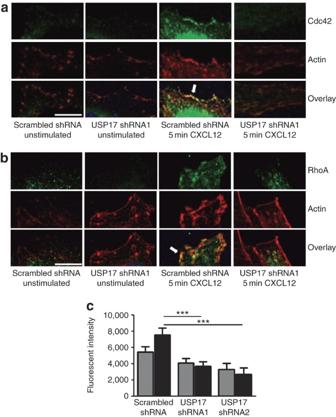Figure 6: GTPase mislocalization at the leading edge by USP17 depletion. HeLa cells were transfected with GFP-tagged Cdc42 (a) or RhoA (b) and either scrambled shRNA or USP17 shRNA1 as indicated. Cells were serum starved and either left unstimulated or stimulated with CXCL12 for 5 min. Cells were then fixed and stained for phalloidin-actin (red) and visualized by confocal microscopy. Scale bar, 10 μm. Arrows indicate areas of actin and GTPase plasma membrane colocalization. (c) HeLa cells were transfected with GFP-tagged RhoA along with either scrambled shRNA or USP17 shRNA1 and cells were serum starved for 12 h before imaging. At least ten brightfield and green TIRF images were captured per condition before and post stimulation with CXCL12 (100 ng ml−1), in triplicate experiments. Fluorescence was scored on the basis of green TIRF per cell; values are mean±s.e.m.; and statistical analyses are relative to scrambled shRNA control by one-way analysis of variance. ***P>0.005. Grey bars indicate unstimulated cells, whereas black bars are CXCL12-stimulated cells. Figure 6: GTPase mislocalization at the leading edge by USP17 depletion. HeLa cells were transfected with GFP-tagged Cdc42 ( a ) or RhoA ( b ) and either scrambled shRNA or USP17 shRNA1 as indicated. Cells were serum starved and either left unstimulated or stimulated with CXCL12 for 5 min. Cells were then fixed and stained for phalloidin-actin (red) and visualized by confocal microscopy. Scale bar, 10 μm. Arrows indicate areas of actin and GTPase plasma membrane colocalization. ( c ) HeLa cells were transfected with GFP-tagged RhoA along with either scrambled shRNA or USP17 shRNA1 and cells were serum starved for 12 h before imaging. At least ten brightfield and green TIRF images were captured per condition before and post stimulation with CXCL12 (100 ng ml −1 ), in triplicate experiments. Fluorescence was scored on the basis of green TIRF per cell; values are mean±s.e.m. ; and statistical analyses are relative to scrambled shRNA control by one-way analysis of variance. *** P >0.005. Grey bars indicate unstimulated cells, whereas black bars are CXCL12-stimulated cells. Full size image Although USP17 depletion induced baseline activation of the GTPases examined, the GTPases did not localize at the plasma membrane. To confirm that the mislocalized GTPases were indeed not able to signal downstream, we examined the activation of various well-characterized proteins normally upregulated when GTPases are membrane activated. Following CXCL12 stimulation when USP17 is depleted, we observed that activation of the downstream effectors PAK, β1 integrin and ERK1/2 was greatly diminished compared with scrambled shRNA-transfected cells ( Fig. 7 ). The finding that there was no increase in activation of effector proteins in USP17-depleted cells is in agreement with the data presented in Figure 5b , demonstrating no upregulation of GTPase activation in USP17-depleted cells. Therefore, USP17 is required for normal membrane localization of active GTPases and the upregulation of downstream signalling pathways following stimulation and consequent cell motility. 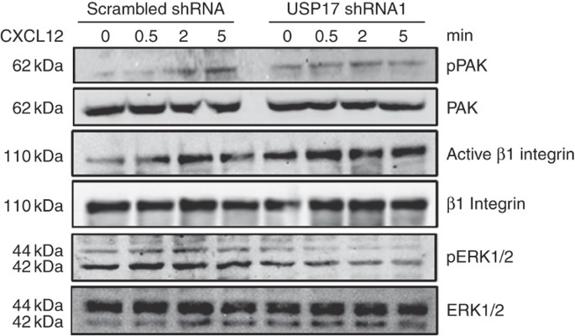Figure 7: USP17 depletion results in blunted downstream signalling. HeLa cells were transfected with either scrambled shRNA or USP17 shRNA1 and stimulated with CXCL12 (100 ng ml−1) for 0, 0.5, 2 or 5 min. Protein was collected and whole-cell lysates were immunoblotted for pPAK, total PAK, active β1 integrin, total β1 integrin, pERK1/2 and total ERK1/2 as indicated. Figure 7: USP17 depletion results in blunted downstream signalling. HeLa cells were transfected with either scrambled shRNA or USP17 shRNA1 and stimulated with CXCL12 (100 ng ml −1 ) for 0, 0.5, 2 or 5 min. Protein was collected and whole-cell lysates were immunoblotted for pPAK, total PAK, active β1 integrin, total β1 integrin, pERK1/2 and total ERK1/2 as indicated. Full size image Deubiquitination enzymes have been demonstrated to be involved in multiple cellular processes [1] . The data presented here represent the first implication of their role in regulating both mesenchymal and amoeboid cell motility. USP17 has been identified as an immediate early gene induced by cytokines [5] , [6] , [8] . However, here we have demonstrated that USP17 is also rapidly induced by chemokines and USP17 expression is required for chemotaxis and chemokinesis, adding to its previously characterized role in cell-cycle progression [8] , [11] . The reduced actin and tubulin polymerization suggests that USP17 is crucial for cell migration and reorganization of the cytoskeleton. The ability of cells to change morphology and type of migration gives them the advantage of movement through various extracellular conditions, thus adapting to environmental constraints. Cell plasticity is well documented in cancer biology [28] and its role in other pathologies such as inflammation has also been appreciated [29] , [30] . Interestingly, cells lacking USP17 have fewer cell protrusions, appear rounded, have decreased cytoskeleton polymerization and have markedly decreased migration distance and rate. As the Rho family of GTPases has been shown to regulate the cytoskeleton and therefore cell motility [22] , [31] , we postulated that inhibiting GTPase membrane localization may be the mechanism of the decreased migration. Indeed, we have previously demonstrated that USP17 is implicated in the mislocalization of Ras GTPase through the regulation of its processing and in particular the modulation of the protease RCE1 (refs 10 , 32 ); here, we illustrate that depletion of USP17 blocked RhoA, Rac1 and Cdc42 membrane localization. These GTPases have been reported to be processed in a similar manner [33] and could indicate that RCE1 regulation is responsible, although it is likely to not be the sole USP17 substrate and other targets may be involved. It is clear, however, that the active Rho GTPases are mislocalized in the absence of USP17 and when combined with the failure to activate their downstream effectors, could explain the defects in cytoskeletal reorganization and migration. RhoA or Rac1 are individually required for mesenchymal or amoeboid migration, respectively; therefore, preventing proper localization of both these GTPases along with Cdc42 would certainly inhibit motility [23] , [24] , [34] . In addition, the Ras GTPases also have a role in cell migration [35] , and we have previously demonstrated that USP17 is also able to regulate H-Ras and N-Ras membrane localization and activation [10] . The ability to modulate Ras and Rho GTPase family members through inhibition of USP17 may be a useful way to block both mesenchymal and amoeboid motility. Interestingly, another DUB CYLD (cylindromatosis gene) has also been suggested recently to regulate cell migration through the GTPase Rac1 (refs 36 , 37 ). It was demonstrated that inhibiting CYLD resulted in decreased migration, which correlated with blunted membrane ruffling, microtubule shortening, decreased polarization and reduced Rac1, but not RhoA or Cdc42 activity. This suggests that CYLD is able to regulate elongated cell motility, but not amoeboid migration. Our results using CYLD as a control demonstrated that CYLD depletion was not required for chemotaxis in our system, likely because these cells will still be able to undergo amoeboid migration. Therefore, CYLD and USP17 have distinct roles in regulating Rho GTPases and cell motility. In summary, our findings show that expression of the DUB USP17 is essential for chemotaxis and chemokinesis, and represents a potential new therapeutic target for regulating pathologies with aberrant cell motility. As our understanding of the function and regulation of these DUBs increases, the ability to target them and prevent disease is promising [38] . Indeed, inhibitors for DUBs such as USP7 are currently in development [39] . Previously, USP17 has been demonstrated to regulate both cell proliferation and G1/S cell-cycle progression and is increased in tumours [11] , [32] . Therefore, the dual role of USP17 in regulating cell growth and migration makes it an ideal candidate for the development of potential inhibitors in these diseases. Plasmids pSUPER-scrambled shRNA and pSUPER-USP17 shRNA1 (target sequence 5′-GCAGGAAGATGCCCATGAA-3′) were kind gifts from Dr Rene Medema (University Medical Center, Utrecht, the Netherlands). pRS-USP17 shRNA2 (target sequence 5′-AAGAGCCACTCAGGAAAGCACCTTAGACC-3′) and pRS-USP17 shRNA3 (target sequence 5′-GATGATTTGGCTCCTGTGGCAAGACAGCT-3′) were purchased from Origene Technologies. pGFP-RS-USP17 shRNA (target sequence 5′-GCAGGAAGATGCCCATGAA-3′) was purchased from Origene technologies. pCAGGS-eGFP-Cdc42, pCAGGS-eGFP-Rac1 and pCAGGS-eGFP-RhoA were kind gifts from Dr Michiyuki Matsuda (Osaka University, Osaka, Japan). pDQ-EV (His), pDQ-USP17 (His) and pDQ-USP17CS (His) were kind gifts from Dr Derek Quinn (Queen's University, Belfast). Cell culture and transfection Hut78 and U937 cells were grown in RPMI 1640 (PAA) and HeLa and MDA-MB-231 cells (American Type Culture Collection, Manassas, USA) in DMEM, supplemented with 10% FCS, 1% penicillin (10,000 U ml −1 )/streptomycin (10,000 μg ml −1 ) and 1% L -glutamine (200 mM), grown at 37 °C in a 5% CO 2 humidified incubator. Hut78 cells were transfected using the Amaxa Nucleofector System (Lonza). U937, MDA-MB-231 and Hela cells were transfected with FuGENE6 (Roche) according to the manufacturer's instructions. For those experiments with CXCL12 or CXCL8 stimulation, cells were rested for 12 h in DMEM without serum, then stimulated with the chemokine for the indicated times and concentrations indicated. Primary cell isolation Whole peripheral blood packs were donated by Northern Ireland Blood Service (Belfast, UK) or peripheral blood was drawn from healthy donors using 0.5 ml of 0.5 M EDTA (pH 8.0) as an anticoagulant. PBMCs and polymononuclear neutrophils (PMNs) from healthy volunteers were isolated from 50 ml of whole blood by density gradient centrifugation at 650 g for 30 min over Ficoll (Amersham). PMNs were isolated by centrifugation and hypotonic lysis of erythrocytes. The cells were then washed twice at 290 g for 10 min with RPMI medium before counting. RT–PCR mRNA was extracted from cells using STAT60 reagent (Biogenesis), and RNA isolation was performed according to the manufacturer's instructions. RT–PCR analysis of 1 μg total RNA was performed using the OneStep RT–PCR kit (Qiagen) according to the manufacturer's instructions, and separated on 1% agarose gels [11] . The primer sets used were USP17 forward 5′-CAGTGAATTCGTGGGAATGGAGGACGACTCACTCTAC-3′ and USP17 reverse 5-AGTCATCGATCTGGCACACAAGCATAGCCCTC-3′, and β-actin forward 5′-GGACTTCGAGCAAGAGATGG-3′ and β-actin reverse 5′-AGCACTGTGTTGGCGTACAG-3′. Immunoprecipitation and immunoblotting Cells were washed once with ice-cold PBS and resuspended in 1% Triton lysis buffer containing protease inhibitors (1 mM Na 3 V0 4, 10 μg ml −1 leupeptin, 10 μg ml −1 aprotinin and 1 mM phenylmethylsulphonyl fluoride). Where indicated, cells were immunoprecipitated using the monoclonal USP17 antibody (Fusion Antibodies). Immunoprecipitations or whole-cell lysates (IB) were separated by SDS polyacrylamide gel electrophoresis, transferred to polyvinylidene difluoride membrane and probed with the appropriate antibodies. Antibodies used are listed in Supplementary Table S1 . Proteins were detected using the enhanced chemiluminescence detection method (Amersham), exposed using the ChemiDoc XRS imaging system (Bio-Rad) and analysed with The Discovery Series software from Quantity One version 4.5.0 (Bio-Rad). GTPase activation pulldowns Cells were washed once with ice-cold PBS and lysed in 200 μl lysis buffer (50 mM Tris-HCl, pH 7.5, 1% Triton X-100, 100 mM NaCl, 10 mM MgCl 2 , 5% glycerol, 1 mM Na 3 VO 4 ) containing protease inhibitors (1 mM Na 3 V0 4 , 10 μg ml −1 leupeptin, 10 μg ml −1 aprotinin and 1 mM phenylmethylsulphonyl fluoride). Cell lysates were incubated at 4 °C for 1 h with GST-fusion protein (GST-PAK for CDC42 and Rac1 of GST-Rhotekin for RhoA) coupled to glutathione-sepharose beads (Amersham Biosciences) as described previously [11] . Protein was run on SDS polyacrylamide gel electrophoresis gels and analysed as indicated in the previous section. Active GTPases and whole-cell lysates were detected by immunoblotting with the appropriate antibodies. Boyden chamber cell migration assay MDA-MB-231 and HeLa cells were plated in 12 mm-diameter Transwells (Corning Costar), transfected with the indicated plasmids and stimulated with 20 ng ml −1 CXCL12 (PeproTech). Plates were then incubated at 37 °C in 5% CO 2 for 20 h. Migrated cells at the bottom of the top chamber were fixed for 10 min in methanol, stained with crystal violet solution (0.05% crystal violet and 25% methanol), washed and air-dried for 1 h. The filters were then destained with cell migration destaining solution (1:1 ethanol: 0.2 M sodium citrate) and measured using a microplate reader read at A 570 . Fixed cell confocal imaging Cells were seeded and transfected on LabTek II, CC2-treated chamber slides as described, fixed in 4% paraformaldehyde for 20 min, permeabilized with 0.5% Triton for 5 min and stained with the indicated antibodies and/or costain, which are listed in Supplementary Table S2 . Slides were viewed using a Leica TCS SP5 DMI6000 CS Confocal Microscope (Leica) using the following lasers: ultraviolet (355 nm), Argon (488 nm) and HeNe (543 nm, 633 nm). Fluorescent images were captured with a 40× lens zoomed in 1–3× with a 1,024×1,024 frame and 400 Hz scanning speed. Images were analysed using Leica LAS AF software (Leica) and ImageJ (NIH). Live cell migration assay Hut78 migration assays were carried out in nunclon 96-well plates. On the evening before the migration, a goat anti-mouse capture antibody (Sigma) was added to the wells and left overnight at 4 °C. Wells were washed and incubated with a mouse anti-CD11a antibody (Monosan Clone SPV-L7) for 3 h at 37 °C. Wells were washed three times, and 10,000 cells per 100 μl were added to the wells and left for 15 min before beginning live cell image capture using the IN Cell Imager 1000 (GE Healthcare). Brightfield images were captured every 60 s for 90 min and images at 480×535 nm were taken at 0 and 90 min and cell migration was measured using ImageJ software (NIH). Alternatively, HeLa cells were plated onto glass-bottomed 35 mM μ-dishes (Ibidi) and transfected as previously described. At 48 h post infection, images were captured every 15 s for 10 min using a Leica TCS SP5 Confocal Microscope and analysed using ImageJ software (NIH). TIRF microscopy HeLa cells were plated onto 35 mM MatTek glass-bottomed dishes (MatTek), and transfected with GFP-tagged RhoA along with scrambled shRNA, USP17 shRNA1 or USP17 shRNA2. At 48 h post transfection, cells were serum starved for 12 h. Brightfield and TIRF images were captured using the Nikon Eclipse Ti both before and after stimulation with CXCL12. TIRF settings were kept at 200 ms exposure and gain 10 and brightfield at 100 ms exposure and gain 10 at 60× magnification. Analysis for Green TIRF fluorescence was performed using NIS Elements AF 3.1 Software. How to cite this article: de la Vega, M. et al . The deubiquitinating enzyme USP17 is essential for GTPase subcellular localization and cell motility. Nat. Commun. 2:259 doi: 10.1038/ncomms1243 (2011).